Thermal conductance of metal–diamond interfaces at high pressure The thermal conductance of interfaces between metals and diamond, which has a comparatively high Debye temperature, is often greater than can be accounted for by two-phonon processes. The high pressures achievable in a diamond anvil cell (DAC) can significantly extend the metal phonon density of states to higher frequencies, and can also suppress extrinsic effects by greatly stiffening interface bonding. Here we report time-domain thermoreflectance measurements of metal–diamond interface thermal conductance up to 50 GPa in the DAC for Pb, Au 0.95 Pd 0.05 , Pt and Al films deposited on type 1A natural [100] and type 2A synthetic [110] diamond anvils. In all cases, the thermal conductances increase weakly or saturate to similar values at high pressure. Our results suggest that anharmonic conductance at metal–diamond interfaces is controlled by partial transmission processes, where a diamond phonon that inelastically scatters at the interface absorbs or emits a metal phonon. Interfaces play a key role in the science and engineering of materials and often determine the performance of engineering systems. Examples span the range from the mechanical properties of composites to the efficiency of photovoltaics to the corrosion of metals. Here we are concerned with the exchange of thermal energy across an interface between two materials. This topic is of great current interest for the development of higher densities of information storage using thermally mediated processes in phase change memories (PCMs) [1] and heat-assisted magnetic recording (HAMR) [2] . Precise control of heat input and spreading is necessary to minimize power demands and write to nanoscale bits of information without corrupting adjacent bits. As there are boundaries between the densely packed bits of memory, understanding thermal conductance across those interfaces is critical for the further development of PCM and HAMR. Gaps in fundamental understanding of the thermal conductance of interfaces, although identified over 20 years ago [3] , persist to this day [4] , [5] . Thermal conductance is an integral property that convolutes contributions from a variety of heat carriers that have spectral distributions in their density, group velocity and dominant scattering mechanisms. A typical experiment measures how much heat is transported across an interface, but not the spectral distribution of the heat current, or the governing mechanisms. The interface between many metals and diamond, however, is a special case where elastic phonon processes clearly comprise only a fraction of the total thermal conductance. The phonon radiation limit [3] , [6] describes the maximum possible thermal conductance for elastic phonon transmission across an interface that is consistent with the respective phonon densities of states (DOS). This elastic limit lies a factor of 5–10 below the measured Au/diamond and Pb/diamond interface thermal conductances [3] , [7] . Inelastic phonon-scattering processes are probably significant at most material interfaces above cryogenic temperatures, but metal–diamond interfaces produce an extreme situation that enables the study of inelastic processes. In addition to advancing the thermal design of PCM, HAMR and other nanoscale devices, understanding metal–diamond thermal conductance has direct relevance to the goal of using diamond as a substrate for high power radio frequency (RF) devices [8] and the thermal performance of diamond–metal composites [9] , [10] . Prior work at ambient pressure has implicated inelastic phonon scattering as the source of the excess metal–diamond conductance. Bi/diamond and Pb/diamond show a linear temperature dependence inconsistent with two-phonon elastic scattering models [7] . In 2009, Hopkins [11] described a model for diamond phonons absorbing or emitting 2–3 identical metal phonons. Duda and colleagues [12] subsequently generalized this model into the so-called anharmonic inelastic model (AIM). The AIM captures the magnitude and temperature dependence of the conductance of metal interfaces with diamond by considering n -phonon processes involving one diamond phonon emitting or absorbing n −1 metal phonons. A recent non-equilibrium molecular dynamics (MD) simulation by Sääskilahti et al . [13] for an Ar:heavy-Ar interface suggests that frequency-doubling and -halving inelastic processes are favoured. That is, the MD simulation suggests the importance of a mechanism where a diamond phonon splits into two equal frequency metal phonons, in support of the AIM model. Aside from inelastic phonon processes, electron–phonon interactions may also play a significant role by either suppressing or enhancing the conductance. Given an adiabatic heat flux boundary condition on metal electrons at a metal–nonmetal interface, a two-temperature model predicts a thermal resistance of in series with the phonon–phonon conductance channel [14] . Here g is the volumetric electron–phonon coupling parameter and Λ L is the lattice thermal conductivity of the metal. Past theoretical work has argued that electron–phonon coupling may alternately increase the conductance, and that the thermal conductance of Au–diamond may have a significant contribution from heat transfer between Au electrons and diamond phonons [15] , [16] , [17] . These models describe an electron–phonon conductance in parallel with the phonon channels, as opposed to a resistance in series. However, these theories are apparently inconsistent with experiments that found that the thermal conductances of Bi and Pb interfaces with diamond are similar even though the electronic heat capacity of Pb is ~600 times that of Bi [3] , [7] . Another consideration is thermal conductance by electrons that are heated far out of equilibrium with the lattice [18] , [19] , [20] . Our experiments utilize metal–diamond cooling rates at the nanosecond timescale, well after the electrons have equilibrated with the lattice. Thermal conductance at an interface can be complicated by surface chemistry and thin layers of interfacial material. To study intrinsic properties, these extrinsic factors should be minimized or controlled. This has motivated experiments on H-terminated diamond [7] , metal–diamond conductances under a range of surface treatments [21] , [22] , [23] , interfacial graphene [24] and self-assembled monolayers [25] . Often, interfacial material produces weak bonding and limits the conductance, which is of interest in itself but obscures other conductance mechanisms involved in the transport of thermal energy across the interface. By applying 12 GPa of pressure to weak Al/SiC interfaces, Hsieh et al . [26] showed that the influence of weak interfacial bonding on the thermal conductance can be reversibly removed. In this paper, we report measurements of metal–diamond interface thermal conductance for Pb, Au 0.95 Pd 0.05 , Pt and Al films deposited on type 1A (nitrogen-rich) natural [100] and type 2A (nitrogen-free) synthetic [110] diamond anvils up to 50 GPa in the diamond anvil cell (DAC). The thermal conductances increase weakly or saturate to similar values at high pressure in all cases. We expect three-phonon processes involving two metal phonons to have a strong pressure dependence, therefore the data suggest that such processes are not dominant, and that the important anharmonic process involves two phonons in diamond and one phonon in the metal. 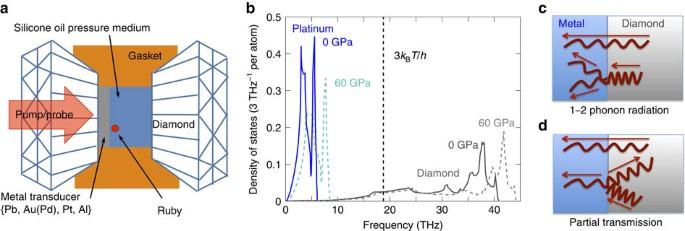Figure 1: Experimental concept. (a) The experimental system, where we use time-domain thermoreflectance (TDTR) to measure the thermal conductance of metal–diamond interfaces at high pressure in a DAC. (b) Illustration of how high pressure stiffens the metal36, increasing its maximum phonon frequency and its overlap with the diamond density of states (DOS)29. (c) Elastic phonon transmission across the interface and two-phonon radiation into the metal. (d) Example of a three-phonon partial transmission (PT) process. Our results provide strong evidence that PT processes control the inelastic conductance across interfaces between materials with low overlap in their phonon DOS. Experiment Figure 1 illustrates our experiment and the underlying concepts. At pressures in the tens of GPa, comparable to the bulk modulus of many metals, the phonon DOS extends to significantly higher frequencies. By measuring different metal films on diamond as a function of pressure, we can explore a wide range of characteristic phonon frequencies in the metals, for a relatively unchanged diamond DOS. Figure 1: Experimental concept. ( a ) The experimental system, where we use time-domain thermoreflectance (TDTR) to measure the thermal conductance of metal–diamond interfaces at high pressure in a DAC. ( b ) Illustration of how high pressure stiffens the metal [36] , increasing its maximum phonon frequency and its overlap with the diamond density of states (DOS) [29] . ( c ) Elastic phonon transmission across the interface and two-phonon radiation into the metal. ( d ) Example of a three-phonon partial transmission (PT) process. Our results provide strong evidence that PT processes control the inelastic conductance across interfaces between materials with low overlap in their phonon DOS. Full size image Time-domain thermoreflectance (TDTR) is a well-established optical pump-probe technique for measuring thermal transport properties [27] . Our TDTR system uses a Ti:sapphire ultrafast pulsed laser with a 785-nm centre wavelength, so the diamond anvils serve as transparent windows to the metal films for our experiment, which we deposited on the diamond anvil culets directly. The pressure is measured using ruby calibrants and the silicone oil Brillouin frequency; see Methods, Supplementary Note 1 and Supplementary Fig. 1 for details. The TDTR measurement and data analysis proceed normally, except that bidirectional heat flow into both the pressure medium and diamond anvil must be taken into account [28] . We obtain the metal–diamond interface thermal conductances by fitting the bidirectional TDTR thermal model to the measured TDTR data. The important thermal parameters, such as the metal film areal heat capacity, are extrapolated to high pressure using known pressure–volume equations of state ( Supplementary Note 2 and Supplementary Fig. 2 ). For the TDTR measurement to have sensitivity to the thermal conductance G between a thin metal film and substrate, the rate at which the metal film surface cools should be limited by the interface decay time τ G = hC / G and not the thermal diffusion time τ diff = h 2 C /Λ in the metal film. Here h , C and Λ are the film thickness, volumetric heat capacity and thermal conductivity, respectively. The condition τ G > τ diff is non-trivial for thick (>100 nm) films of low thermal conductivity metals such as Pt and Pb. To obtain Λ, we applied the Wiedemann–Franz law from four-point probe electrical resistivity measurements at ambient, and found Λ=33, 79, 46 and 150 W m −1 K −1 for our Pb, Au(Pd), Pt and Al films, respectively. τ diff can be nearly 500 ps for the case of 100 nm Pb at zero pressure, since C =1.47 × 10 6 J m −3 K −1 . However, the raw TDTR data show progressive shortening of τ diff with pressure, and we do not observe τ G shorter than 1 ns for the Pt and Pb data sets, where τ diff is longest due to lower Λ. We do not report diamond thermal conductivity data as a function of pressure due to low signal to noise, as discussed in Supplementary Note 3 . At ambient pressure, the conductivity of one of our Al-coated type 1A diamond anvils was ~550 W m −1 K −1 due to nitrogen defects. Multiple measurements with Al and Pt transducers on the type 2A diamond anvil yielded conductivities between 2,200 and 3,400 W m −1 K −1 . The corresponding apparent type 1A and type 2A diamond thermal conductivities with an Au(Pd) transducer were ~400 and 1,100–1,500 W m −1 K −1 at ambient pressure. These fitted values for the type 2A diamond, and the difference between Al, Pt and Au(Pd) values, should not be taken as quantitative measurements of the thermal conductivity of type 2A diamond. The measurement sensitivity and signal to noise for this parameter is low, the high reflectivity of Au(Pd) exacerbates the low signal to noise, and the bulk thermal conductivity of diamond does not decrease because Au(Pd) is coating its surface instead of Al. With the Pb transducer, the interface conductance at 0 GPa was too low for appreciable sensitivity to the diamond thermal conductivities. Regardless, the thermal conductivity measured by TDTR occurs in the bulk of the diamond at the timescale of the 9.8-MHz pump modulation frequency. Thermal transport at that timescale is not relevant to conductance across the metal–diamond interface, which occurs in the sub-10-ns regime. 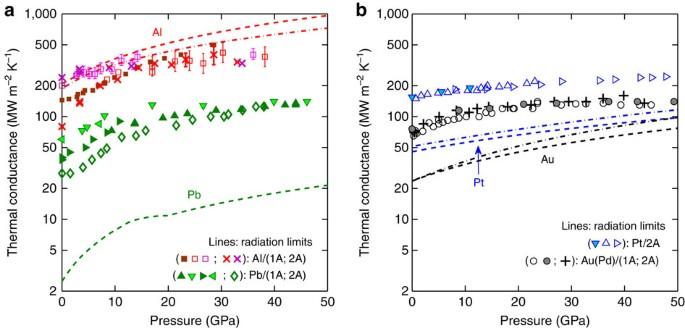Figure 2: Metal–diamond interface thermal conductances. The thermal conductances of Al, Pt, Au(Pd) and Pb on type 1A [100] and type 2A [110] oriented diamond anvils were measured as a function of pressure in the DAC by time domain thermoreflectance (TDTR). The results are separated intoa,bfor ease of viewing. The data and radiation limits (dashed lines) are colour coded: red hues for Al, blue for Pt, black for Au(Pd) and green for Pb. The dot-dashed lines are alternative radiation limits using theoretical phonon cutoff frequencies from the literature (Fig. 3). Magenta symbols, downward filled cyan triangles, filled grey circles and left/down-facing bright green triangles are decompression data for Al, Pt, Au(Pd) and Pb, respectively. The kink in the Pb radiation limit from 13–20 GPa is from an interpolation across the broad phase transition between face-centered cubic (fcc) and hexagonal close-packed (hcp) Pb in that pressure range (Supplementary Note 2). The error bars on certain high pressure Al points represent random uncertainty in the TDTR thermal model fits, owing to a reduced thermoreflectance signal from Al at high pressure (Supplementary Fig. 3). Not shown is ≈±15% systematic uncertainty due to uncertainty in the extrapolation of the metal film areal heat capacity (Supplementary Note 3). Interface thermal conductance Figure 2a,b shows all of the high pressure metal–diamond thermal conductance data. The results for Al and Pb, and for Pt and Au(Pd), are split into separate figures for clarity. Data are colour coded by the metal transducer: red hues belong to Al, blue to Pt, black to Au(Pd) and green to Pb. Data are further identified by symbol, as listed in the legend. Magenta symbols, downward filled cyan triangles, filled grey circles and left/down-facing bright green triangles are decompression data for Al, Pt, Au(Pd) and Pb, respectively. Figure 2: Metal–diamond interface thermal conductances. The thermal conductances of Al, Pt, Au(Pd) and Pb on type 1A [100] and type 2A [110] oriented diamond anvils were measured as a function of pressure in the DAC by time domain thermoreflectance (TDTR). The results are separated into a , b for ease of viewing. The data and radiation limits (dashed lines) are colour coded: red hues for Al, blue for Pt, black for Au(Pd) and green for Pb. The dot-dashed lines are alternative radiation limits using theoretical phonon cutoff frequencies from the literature ( Fig. 3 ). Magenta symbols, downward filled cyan triangles, filled grey circles and left/down-facing bright green triangles are decompression data for Al, Pt, Au(Pd) and Pb, respectively. The kink in the Pb radiation limit from 13–20 GPa is from an interpolation across the broad phase transition between face-centered cubic (fcc) and hexagonal close-packed (hcp) Pb in that pressure range ( Supplementary Note 2 ). The error bars on certain high pressure Al points represent random uncertainty in the TDTR thermal model fits, owing to a reduced thermoreflectance signal from Al at high pressure ( Supplementary Fig. 3 ). Not shown is ≈±15% systematic uncertainty due to uncertainty in the extrapolation of the metal film areal heat capacity ( Supplementary Note 3 ). Full size image Decompression (decreasing pressure) is distinguished from compression (increasing pressure) because of hysteresis, where the decompression conductances are generally higher but limited by the maximum conductance reached. The red/magenta and filled brown squares represent two different Al films on the same type 1A diamond anvil, and similarly for the right/left and up/down triangle pairs for Pb on type 1A diamond. The compression runs on separate Au(Pd) films are not distinguished. The Pt on type 2A data is from three separate pressure runs on the same Pt film; it was decompressed twice. The error bars on selected Al points represent random uncertainty in the fitted conductance owing to low signal levels from Al at high pressure ( Supplementary Note 4 and Supplementary Fig. 3 ). Not shown is the roughly ±15% systematic uncertainty propagated from our high pressure extrapolations of relevant TDTR thermal model parameters ( Supplementary Note 3 ). One-phonon radiation limit The dashed lines in Fig. 2a,b are one-phonon radiation limits for the respective metals on diamond [3] . The one-phonon radiation limit is the maximum thermal conductance achievable in a two-phonon process, that is, the interaction of one phonon in diamond with one phonon in the metal layer. It assumes that all diamond phonons with ω < ω c that impinge on the interface transmit, where ω c is the maximum (cutoff) phonon frequency in the metal. For low cutoff frequency metals such as Au(Pd) and Pb in contact with diamond, the high-temperature Debye approximation is valid. Here v d is the diamond Debye velocity: , where v l and v t are the longitudinal and transverse sound velocities in diamond, respectively. This simplification is not well satisfied for higher cutoff frequency metals Pt and Al, particularly at high pressure, so we instead apply a finite temperature radiation limit, starting from equation (16) of ref. 3 : Here the sum over j is over the diamond phonon modes, the superscript B indicates the sum is over phonons moving towards the interface, n ( ω , T ) is the thermal occupation, d ω j /d k is the diamond group velocity, D ( ω ) is the phonon DOS and t ( ω ) is the transmission coefficient, which is assumed in the radiation limit model to be unity for ω ≤ ω c and zero otherwise. To approximate the diamond group velocities and DOS as a function of pressure, we assume an isotropic quadratic dispersion in the longitudinal and transverse acoustic modes, as opposed to the linear Debye model. The pressure dependence of the acoustic mode parameters are taken by linear interpolation between best isotropic fits to the diamond dispersions at 0 and 50 GPa (ref. 29 ). These dispersion relations are then used to compute the group velocities and DOS. The diamond optical modes are irrelevant, since they are always above the metal cutoff frequencies. In the end, using a quadratic rather than linear dispersion only increases the radiation limit slightly. The quadratic dispersion contains opposing corrections: higher DOS and lower group velocities in the acoustic modes near the Brillouin zone edge. The ω c for the metals are assumed to scale linearly with the Debye temperature of the metal, which increases with pressure according to T D = T D,0 [ K T / K T,0 ] 1/2 [ V / V 0 ] 1/6 . Here K T =− V d P /d V and V / V 0 come from the respective pressure–volume equations of state for Au [30] , Pb [31] , [32] , Pt [33] and Al [34] . 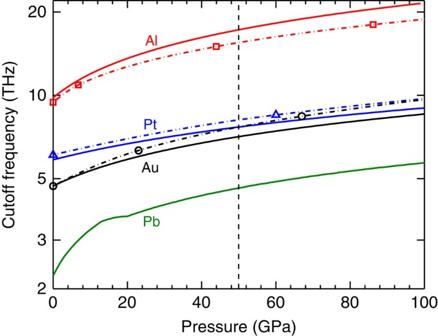Figure 3: High pressure cutoff frequencies. We extrapolate the maximum or cutoff frequenciesωcfor Al, Pt, Au and Pb phonons based on a linear scaling with the Debye temperature itself derived from the pressure–volume EOS of the metals (Supplementary Note 2). This extrapolation is in fair agreement with prior theoretical results for Al, Pt and Au (points and dot-dash lines)35,36,37. At 50 GPa, our Debye extrapolation deviates from the theoreticalωcof Al, Pt and Au by +11%, −6% and −8%, respectively. Figure 3 shows the resulting ω c and compares them to more sophisticated theoretical and first-principles calculations for Al [35] , Pt [36] and Au [37] . At 50 GPa, our Debye extrapolation deviates from the theoretical ω c of Al, Pt and Au +11%, −6% and −8%, respectively. Since the radiation limit scales strongly with ω c , our G 1R at 50 GPa differ by +32%, −16% and −21% from radiation limits calculated with the theoretical ω c . We expect comparable error in our extrapolated Pb ω c at the highest pressures. Figure 3: High pressure cutoff frequencies. We extrapolate the maximum or cutoff frequencies ω c for Al, Pt, Au and Pb phonons based on a linear scaling with the Debye temperature itself derived from the pressure–volume EOS of the metals ( Supplementary Note 2 ). This extrapolation is in fair agreement with prior theoretical results for Al, Pt and Au (points and dot-dash lines) [35] , [36] , [37] . At 50 GPa, our Debye extrapolation deviates from the theoretical ω c of Al, Pt and Au by +11%, −6% and −8%, respectively. Full size image The quantity G − G 1R ( Fig. 4 ), when positive, represents the minimum value of the thermal conductance that is not due to elastic phonon processes, within the uncertainty in our extrapolation of G 1R to high pressure. Negative values for G − G 1R imply that anharmonic phonon processes are not necessary to describe the total conductance. If we posit electron–phonon resistance ( Supplementary Note 5 and Supplementary Fig. 4 ), the ‘phonon-only’ G pp − G 1R for Au(Pd) and Pb may be roughly 20–30% higher, closer to the Pt values. 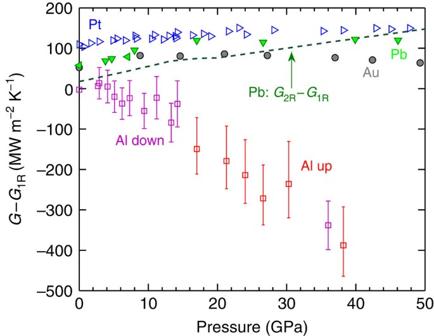Figure 4: Excess thermal conductance. The remainderG−G1Rrepresents the minimum value of the thermal conductance that is not due to elastic phonon processes.G1Ris calculated from our Debye extrapolated cutoff frequencies and not from the theoretical cutoff frequencies from the literature (Fig. 3). We only include data fromFig. 2a,bthat represent the intrinsic thermal conductance in the absence of weak interfacial bonding. The open blue triangles for Pt include all the Pt data, the red squares are for Al on compression (‘Al up’) and the rest are Pb, Au(Pd) and Al decompression data. The dark green dashed line isG2R−G1R≈7 ×G1Rfor Pb. It shows that for Pb,G(P) is comparable to its two-phonon radiation limitG2R. This is not the case for Pt or Au(Pd). Figure 4: Excess thermal conductance. The remainder G − G 1R represents the minimum value of the thermal conductance that is not due to elastic phonon processes. G 1R is calculated from our Debye extrapolated cutoff frequencies and not from the theoretical cutoff frequencies from the literature ( Fig. 3 ). We only include data from Fig. 2a,b that represent the intrinsic thermal conductance in the absence of weak interfacial bonding. The open blue triangles for Pt include all the Pt data, the red squares are for Al on compression (‘Al up’) and the rest are Pb, Au(Pd) and Al decompression data. The dark green dashed line is G 2R − G 1R ≈7 × G 1R for Pb. It shows that for Pb, G ( P ) is comparable to its two-phonon radiation limit G 2R . This is not the case for Pt or Au(Pd). Full size image The green line represents ( G 2R − G 1R ) Pb , which is the amount by which the Pb/diamond two-phonon radiation limit exceeds the one-phonon radiation limit. Analogous to G 1R , G 2R is the upper limit on conductance for three-phonon processes involving one diamond phonon, which we discuss in the next section. It is included for comparison because fourth- and higher-order phonon processes have been considered for the Pb/diamond interface in the past [12] . The two-phonon radiation limits for Au(Pd) and Pt have much higher values, starting >150 MW m −2 K −1 at ambient and increasing rapidly with pressure. While the radiation limit is just an upper bound on the elastic conductance, we have reason to believe it is a good approximation to the elastic conductance across highly mismatched interfaces. In such cases, the diffuse mismatch model and radiation limit predictions are very similar, since the diffuse mismatch model transmission coefficient into the low frequency material is already near unity. Prior work found that the thermal conductance of Pb/Si and Bi/Si interfaces scale with their radiation limits at low temperature to within a factor of 2 (ref. 7 ). In another work, the thermal conductance between Fe-doped rhodium and sapphire was found to converge to its radiation limit <50 K (ref. 38 ). At low temperatures, the phonons above the cutoff of the lower frequency material are partly frozen out, which reduces the inelastic contribution to the thermal conductance and tends to reveal the elastic channel. Three-phonon-scattering models The two-phonon radiation limit is an extension of the one-phonon radiation limit that allows diamond phonons up to twice the metal cutoff frequency to participate. In the high-temperature Debye model, the two-phonon radiation limit is simply G 2R =8 G 1R . Both radiation limits have a strong pressure dependence because the number of diamond phonons that can participate is determined by the metal cutoff frequency. However, the two-phonon radiation limit is restricted to three-phonon processes involving two metal phonons, so now we consider the pressure dependence of three-phonon processes involving just one metal phonon. In the radiation limit, incident diamond phonons with energies E > ℏ ω c are elastically reflected from the interface. We propose that some of these high-energy diamond phonons inelastically scatter at the interface, emitting or absorbing a metal phonon in what we refer to as a partial transmission (PT) process. Since any diamond phonon can participate in PT, this category of phonon interactions at the interface has a large phase space. We write the PT thermal conductance as: Here ω d, j is the cutoff frequency for the j th diamond branch, and is the average energy emitted into the metal by a reflecting diamond phonon. In other words, represents the probability that an incident diamond phonon of energy ω j emits a metal phonon of energy ω ′. The lower bound of the ω j integrals are set by the metal cutoff frequency for consistency with the one-phonon radiation limit. We do not know the form of ; we expect that its derivation would require knowledge of bond anharmonicity at the interface [39] . However, a reasonable assumption is that the pressure dependence of ‹ E m › will scale with the average energy of a phonon in the metal, which in the Debye model is (3/4) ℏ ω c . By this assumption, This expression should be an upper bound on the pressure dependence for PT because we expect the factors that we neglected in , the diamond DOS and interface anharmonicity that drives three-phonon processes, to both decrease with pressure. In the high-temperature limit, for ( ω c / ω d ) 2 ≪ 1, , in contrast to the two-phonon radiation limit . The weak pressure dependence of G PT versus G 2R is owing to the fact that diamond phonons contributing to G PT are independent of the metal cutoff frequency, and ω d is relatively insensitive to pressure. To take a specific example, let us assume that PT completely accounts for the extra conductance that we observe in our experimental data for Pt on diamond ( Fig. 4 ). If we assume that all incident diamond phonons above the metal cutoff frequency participate in PT, then we can solve for ‹ E m › in equation (2) by setting G PT ≈100 MW m −2 K −1 . The result is ‹ E m ›=2.4 meV, which is only 13% of the average energy ‹ E m ›=(3/4) ℏ ω c that we assumed earlier. We can remove the Debye energy assumption by instead taking ‹ E m › as the first moment of the Pt phonon energy DOS. For ambient Pt, Feldman and Horton [40] measured ℏ ‹ ω 1 ›=(3/4) k B Θ, where Θ≈245±5 K. So ‹ E m ›≈15.8 meV at zero pressure. In other words, the extra conductance can be fully explained if all incident diamond phonons participate with an average emitted energy of 2.4 meV, or alternately if 15% of incident diamond phonons above the metal cutoff frequency participate with an average emitted energy given by the first moment of the Pt phonon DOS. Similar participation rates on the order of 10% can account for the extra Pt, Au(Pd) and Pb conductances at high pressure as well. To check that PT processes can realistically represent the extra conductance in Fig. 4 , we reformulate G PT in terms of a relaxation time model. The energy flux across the interface is driven by diamond phonons that are out of equilibrium with the metal reservoir. From the relaxation time approximation to the Boltzmann transport equation, we write d E /d t =( ℏ ω / τ )[ n ′− n ( T )]. For a small deviation from equilibrium, n ′= n ( T )+(∂ n /∂ T )Δ T , so d E /d t ≈( ℏ ω / τ )(∂ n /∂ T )Δ T . This defines a volumetric energy transfer rate and relaxation time τ for conductance by PT processes. Integrating g over an interfacial thickness a 0 , we obtain a conductance: We now assume that τ is an average value, so that τ and a 0 can be moved out of the integral, leaving an integral over the diamond heat capacity. Then, G PT = a 0 C /(2 τ ), where C =1.81 J m −3 K −1 at ambient. For an interface region of one metal lattice spacing thick, a 0 ≈0.4 nm, and G PT ≈100 MW m −2 K −1 , it follows that the average relaxation time is τ ≈4 ps. The simple expression Λ=(1/3) Cv 2 τ implies, for diamond with Λ=2,400 W m −1 K −1 and Debye velocity v ≈1.4 × 10 4 m s −1 , that the bulk average anharmonic scattering time in diamond is 20 ps. In other words, the magnitude of the measured Pt/diamond conductance is consistent with a three-phonon-scattering rate near the interface that is only five times higher than in the bulk. The difference may be largely due to anharmonicity of the interfacial bonds and relaxed selection rules for scattering at the interface [39] . While Hsieh et al . [26] observed reversible stiffening of their Al/SiC interfaces up to 12 GPa, we observe that the Al/diamond and Pb/diamond conductances return to significantly higher zero-pressure conductances after decompression. The type 1A diamond was heat cleaned in vacuum before Al deposition, the type 2A surface was not, but both returned to the same conductance on decompression. We deposited Al on the type 2A surface after heat cleaning and measured a 240-MW m −2 K −1 interface conductance, equivalent to the conductances for decompressed Al on diamond. Evidently, by applying over 30 GPa of pressure, we have irreversibly changed the interfacial bonding. Weak interfaces are often caused by organic contaminants; past studies have shown that 1–30 GPa of pressure can drive chemical reactions or polymerization in organic materials [41] . We believe that the decompressed conductances measured in this study are near the intrinsic zero-pressure metal–diamond conductances, in the sense that weak bonding is absent. Thus, for a well-bonded Pb/diamond interface, we may expect a thermal conductance near 60 MW m −2 K −1 at room temperature, twice the value for thermally evaporated Pb/H/diamond [7] and comparable to Au(Pd) on diamond. See Supplementary Note 6 for further discussion. As discussed in the introduction, a two-temperature model predicts a thermal resistance of in series with the phonon–phonon conductance channel [14] . Here g is the volumetric electron–phonon coupling parameter and Λ L is the lattice thermal conductivity of the metal. These G ep would act as resistors in series with the phonon–phonon conductances G pp , such that the measured G would be suppressed from G pp by a factor of ≈1− G / G ep . We calculate that the ambient electron–phonon conductances are ~1,440, 2,800, 250 and 260 MW m −2 K −1 for Al, Pt, Au and Pb, respectively, ( Supplementary Note 5 ). On decompression, we found that the stiffened interface conductances for Al, Pt, Au(Pd) and Pb were approximately 220, 155, 70 and 60 MW m −2 K −1 , yielding electron–phonon suppression factors of ~15%, 5%, 30% and 20%, respectively. We also estimate the pressure scaling of G ep ( Supplementary Fig. 4 ), and estimate that the suppression factor for Al decreases with pressure, and for Au(Pd) and Pb it is insensitive to pressure. If electron–phonon coupling resistance is present, then the underlying G pp for Au(Pd) and Pt are even more similar than the G that we measure. Regardless, the conductances that we measure for Au(Pd) and Pt ( Fig. 2b ) are similar to within a factor of 2. Pt and Au(Pd) have very different band structures, and Pt has an order of magnitude larger electronic DOS near the Fermi energy. It seems difficult to reconcile our data with models of added conductance that depend on electronic properties of the metal. In prior work, we have posited that a significant portion of the interfacial thermal resistance measured in a TDTR experiment can be owing to a spatial mismatch in the spectral distribution of the heat current [42] . If the majority of the heat carried across the interface is carried by different phonons than the phonons that carry heat in the solid, the measured interfacial conductance will include an additional non-equilibrium thermal resistance, . quantifies the resistance between the phonons that carry the heat across the interface and the phonons that carry the heat in the solid, and is analogous to the interfacial electron–phonon resistance. If is an important contributor to the interface conductance values that we measure between Al/Pt/Au/Pb and diamond, then changing the spectral distribution of the diamond thermal conductivity should alter the measured interface conductance. Recent work by Katcho et al . [43] used an ab initio Green’s function approach to calculate the effect of nitrogen defects on the thermal conductivity of diamond. They found that nitrogen defects strongly scatter a broader range of phonons than previously thought, from high frequencies to as low as 5 THz. If the transmission spectrum for heat entering diamond were elastic, much of the heat from Au(Pd) and Pb would enter below 5 THz, and the details of defect scattering >5 THz would not impede transport away from the interface. Since the thermal conductances of Pt, Au(Pd) and Pb on diamond greatly exceed their respective phonon radiation limits, we know the transmission spectrum cannot be mainly elastic for these metals. For Al/diamond, even if the conductance were elastic, the high Al cutoff frequency is within the nitrogen scattering regime in diamond. Ultimately, for non-equilibrium resistance, it does not matter how heat enters the diamond, so much as in which diamond modes the heat enters. Hence, phonons from the metal may be in different degrees of non-equilibrium with heat-carrying diamond phonons near the interface, depending on the presence or absence of nitrogen defect scattering. To check this, we measured metal–diamond thermal conductances on both type 1A (1,500 p.p.m. nitrogen; see Methods section) and type 2A (nitrogen-free) diamond anvils. At pressures high enough to stiffen weak interfacial bonding, we cannot resolve a difference in the interface conductance for the two types of diamond ( Fig. 2a,b ). This suggests that is not an important contributor to the interface conductance. If electron–phonon interactions and non-equilibrium resistance do not control the Al, Pt, Au(Pd) and Pb thermal conductances on diamond, and two-phonon processes cannot produce the observed Pt, Au(Pd) and Pb conductances, then we are left with higher order phonon processes to explain the measured conductances. Three-phonon processes involving two metal phonons should depend strongly on the metal phonon DOS, because only diamond phonons below twice the metal cutoff can participate. However, the Al, Pt, Au(Pd) and Pb DOS encompass a wide range from 0 to 50 GPa, and we do not observe strong pressure or metal cutoff frequency dependence in the conductances, beyond what can be expected from two-phonon processes. This observation at first appears inconsistent with the recent non-equilibrium MD work by Sääskilahti et al . [13] , but we believe that this is because we are studying different systems from different perspectives. Sääskilahti et al . [13] categorized ‘evanescent dissipation’ as part of the elastic thermal conductance in their calculations, whereas we consider it effectively a three-phonon process. This is important because their evanescent component is comparable to their inelastic category, which they calculate is dominated by frequency-doubling or -halving, essentially diamond phonons splitting into multiple equal metal phonons. The other key difference is that Sääskilahti et al . [13] simulated a Ar:heavy-Ar interface with cutoff frequencies of 2 and 1 THz, respectively. We are studying diamond:metal interfaces with cutoff frequency mismatches much >2:1. By analogy we have ‘light-Ar’: heavy-Ar with >2 THz phonons that cannot participate in frequency-halving transmission into the 1-THz material. Such phonons can, however, have evanescent dissipation into the metal. Since the diamond:metal mismatch is several times larger than Ar:heavy-Ar, the phase space for evanescent or PT processes is much larger. Thus, it is not surprising that they dominate over multiple metal–phonon processes in our system. The emphasis of our research is experimental; our models are admittedly approximate and are intended to provide context for our experimental results and physical insight on important thermal conductance mechanisms. The essence of our three-phonon conductance models lie in their pressure dependence. Regardless of the details of the model, for processes involving two metal phonons and one diamond phonon, the conductance must be sensitive to the metal cutoff frequency. This demands a strong pressure dependence that we do not observe. For processes involving two diamond phonons, the pressure dependence is weak because diamond phonons above the metal cutoff frequency can participate. The upper frequency limit to the thermally excited phonons in diamond is 3 k B T / ℏ , and that frequency is independent of pressure. Our null result for non-equilibrium resistance is also consistent with dominant PT. We expect that most diamond phonons gain or lose only a small amount of energy to the metal phonon, so the diamond phonons near the interface should maintain a thermal distribution. In addition, we estimated (equation (4)) that the effective anharmonic scattering rate is ~5 times larger near the interface than in the bulk diamond. A faster scattering rate implies stronger coupling between diamond modes near the interface. Thermal equilibrium, plus enhanced coupling, would tend to suppress any non-equilibrium behaviour in the near-interface region. To summarize, we experimentally show that the metal–diamond interface conductances for Al, Pt, Au(Pd) and Pb increase weakly or saturate at high pressures, that the conductances of Pt, Au(Pd), and Pb on diamond are all of similar magnitude at high pressure and that there is no resolvable distinction in the high pressure conductances for type 1A [100] versus type 2A [110] diamond. We find that compression >above 30 GPa irreversibly stiffens weak interfacial bonding, such that the decompressed metal–diamond conductances are near their corresponding ‘clean interface’ zero-pressure values, ≈60 MW m −2 K for Pb/diamond. The similarity in thermal conductances for Pt and Au(Pd) to high pressure, despite the major differences in their electronic band structures, is difficult to reconcile with existing models of electron–phonon conductance across metal–dielectric interfaces, that is, a contribution to the conductance generated by the coupling of electrons in the metal with phonons in diamond that enhances thermal transport across the interface. For metals with low phonon cutoff frequencies, the extra conductance above the one-phonon radiation limit is likely controlled by PT three-phonon processes, where reflecting diamond phonons emit or absorb a fraction of their energy as a metal phonon. Our calculations indicate that the extra conductance can be accounted for by PT processes with a diamond phonon participation rate ~10%, or alternately, with an interfacial scattering rate ~5 times faster than the three-phonon-scattering rate in bulk diamond at ambient pressure. Thin-film deposition Thin metal films with thicknesses of ≈100 nm were deposited on the culet of either a type 1A or type 2A diamond anvil. Multiple films of Pb, Au 0.95 Pd 0.05 , Pt and Al on diamond were measured by TDTR up to 30–50 GPa and back to ambient pressure. The Au 0.95 Pd 0.05 , Pt and Al films were deposited by direct current (DC) magnetron sputtering. We use Au(Pd) instead of pure Au because Au(Pd) yields a clear picosecond acoustic signal from which we can extract the Au(Pd) film thickness in situ , unlike Au [44] . We measured the Pd content by Rutherford backscattering spectroscopy (RBS) on an Au(Pd)/Si reference. For Al on type 1A diamond and Pt on type 2A diamond, the diamond surface was heated under vacuum before sputtering. The graphite stage, on which the tungsten carbide seat and diamond rested in the vacuum chamber, was resistively heated to ≈650 °C for 10 min and left to cool for 30 min, at which point the Al or Pt was deposited. The standard epoxy fixing the diamond to the carbide seat is heat sensitive, so a strong bond was maintained by sealing the epoxy under a ceramic adhesive. The Pb films were thermally evaporated from a Mo boat using 99.999% Pb shot from Kurt Lesker Inc. in a separate chamber with a base pressure of at most 3 × 10 −7 Torr. The chamber did not have stage-heating functionality as did our sputtering chamber, so instead we pre-heated the seat and diamond anvil assembly in an air furnace to 500 °C for 30 min, removed at 500 °C and loaded it in the evaporation chamber within 10 min. Since Pb films rapidly roughen by de-wetting from diamond if left at or above room temperature, the Pb deposition was done on a liquid nitrogen cooled stage. A type K thermocouple was fed into the chamber to monitor the temperature of the carbide seat, on which the diamond was mounted with ceramic adhesive. During the Pb evaporation, the seat temperature was at or above −90 °C, and at no point did the temperature of the seat fall below −110 °C, as that approaches the frost point of 3 × 10 −7 Torr of water vapour [45] . The Pb/diamond samples were kept in a vacuum desiccator placed in a freezer to halt oxidation and thermally driven de-wetting of the Pb from the diamond until immediately before anvil cell loading. Diamond anvil cell We use a DAC to apply high pressure to the metal–diamond interfaces [46] . The diamond anvils have 400 μm culets with bevels extending to 450 μm. The sample chamber is sealed by a rhenium gasket pre-indented to 50–100 μm with a 200-μm aperture. The pressure medium is 1 cSt viscosity silicone oil (octamethyltrisiloxane, molecular weight 237) from Alfa Aesar or Sigma-Aldrich. Measurements on Au(Pd) and Pb on type 1A diamond were done with the Alfa Aesar silicone oil, all subsequent measurements with the Sigma-Aldrich silicone oil. The Alfa Aesar silicone oil and argon are comparably hydrostatic up to 64 GPa (ref. 47 ), and we observed no significant difference in the performances of the two silicone oils. Except for the Pt data series, where the same Pt film was measured for three DAC loadings, a new metal film was deposited on the same diamond anvil in the same DAC for each loading, and multiple loadings were done for each of the Al, Au 0.95 Pd 0.05 and Pb data series. Between loadings, an ≈20-μm SiC microtool was used to scrape off press-fitted rhenium and the preceding metal film sample, followed by wiping with a cotton swab infused with acetone. This process was repeated until no features are visible on the culet through a stereomicroscope. The following two types of diamond anvils were used: type 1A natural with [100] normal to the culet surface and yype 2A synthetic with [110] orientation. For type 1A, the predominant defects are A- and B-type nitrogen centres, which are arrangements of nitrogen substitutions and vacancies in the diamond lattice [48] . We measured the nitrogen defect content of one of our type 1A anvils by Fourier transform infrared and estimate ~1,500 p.p.m. A- and B centres in total [49] , [50] . This is consistent with the 700-W m −1 K −1 thermal conductivity we measured by TDTR from that type 1A anvil [51] . The thermal conductivities of the type 1A anvils used in this paper varied from 600 to 800 W m −1 K −1 . A type 2A diamond has no nitrogen defects detectable by Fourier transform infrared. At ambient pressure, multiple measurements with Al and Pt transducers yielded type 2A diamond conductivities between 2,200 and 3,400 W m −1 K −1 . The lower end of this range is typical for low-nitrogen diamond with natural isotopic variation [51] . The large scatter is due to a low out-of-phase signal ( Supplementary Note 3 ). Pressure calibration One to three ruby spheres were included in the DAC sample chamber for pressure calibration by ruby fluorescence [52] . The ruby fluorescence shift can be sensitive to non-hydrostatic behaviour of the pressure medium, but the range of variations is small below 50 GPa (ref. 53 ). We estimate ±0.5 GPa uncertainty in the ruby pressure from spectrometer resolution and quasi-hydrostatic effects [54] . One of the Pt/diamond pressure runs (right-facing blue open triangles; Figs 2b and 4 ) was done without ruby spheres. Instead, we calibrated the pressure using an empirical fit f ( P )=13 × P 0.363 to the Brillouin frequency data we obtained from accumulated silicone-side TDTR measurements from other pressure runs ( Supplementary Note 1 and Supplementary Fig. 1 ). The Brillouin calibration measures the pressure precisely where the TDTR measurement is taken [55] , [56] , [57] . The scatter in the f ( P ) data is larger than the statistical error of its points because the rubies are necessarily some distance away from the TDTR measurement point, and the quasi-hydrostatic medium supports small pressure gradients. We estimate ±2 GPa uncertainty in the Brillouin calibration at higher pressures, where our calibration data are sparse. How to cite this article: Hohensee, G. T. et al . Thermal conductance of metal–diamond interfaces at high pressure. Nat. Commun , 6:6578 doi: 10.1038/ncomms7578 (2015).